Electrically tunable optical polarization rotation on a silicon chip using Berry’s phase The continued convergence of electronics and photonics on the chip scale can benefit from the voltage control of optical polarization for applications in communications, signal processing and sensing. It is challenging, however, to electrically manipulate the polarization state of light in planar optical waveguides. Here we introduce out-of-plane optical waveguides, allowing access to Berry’s phase, a quantum-mechanical phenomenon of purely topological origin. As a result, electrically tunable optical polarization rotation on the chip scale is achieved. Devices fabricated in the silicon-on-insulator material platform are not limited to a single static polarization state. Rather, they can exhibit dynamic tuning of polarization from the fundamental transverse electric mode to the fundamental transverse magnetic mode. Electrical tuning of optical polarization over a 19 dB range of polarization extinction ratio is demonstrated with less than 1 dB of conversion loss at infrared wavelengths. Compact system architectures involving dynamic control of optical polarization in integrated circuits are envisioned. Silicon photonics is promising for future highly integrated electronic–photonic systems on the chip scale [1] . In microelectronic integrated circuits, charge carriers utilize metal interconnects, whereas in photonic integrated circuits, photons are guided in optical waveguides. Guided optical waves exhibit inherent properties including amplitude, phase, frequency, wavelength and polarization. Chip-scale silicon strip waveguides are strongly polarization dependent at infrared wavelengths because of the high refractive index contrast to silicon dioxide and the sub-micrometer light confinement [2] . Consequently, the waveguides exhibit large polarization mode dispersion, polarization dependent loss, and polarization dependent wavelength characteristics. While operation in a single-polarization state has been demonstrated to be effective for communications, signal processing and sensing [3] , [4] , [5] , the lack of dynamic polarization control is a significant lacuna in the technology. Electrical control of optical polarization would create new avenues, including routes to advances in modulation [6] , [7] , [8] , [9] , coherent communications [10] , quantum computing [11] , [12] and polarization diversity [13] , [14] . Achieving on-chip polarization control has proven to be elusive. A number of devices and architectures designed to rotate optical polarization have been proposed. Approaches include asymmetric gratings, waveguides with asymmetric slanted sidewalls, dual core waveguides with asymmetric axes, waveguides with asymmetric trenches, triple waveguide couplers and bilayer slots [15] , [16] , [17] , [18] , [19] , [20] . These current methods to realize polarization rotation in silicon suffer from several drawbacks. First, they are static, in the sense that they rotate the polarization by only a fixed amount. Second, they rely on asymmetric geometries with impedance mismatches resulting in degradation of insertion loss. And third, they exhibit wavelength-dependent loss because they rely on periodic structures or mode coupling. To overcome these challenges, we propose and demonstrate chip-scale polarization rotation utilizing Berry’s phase [21] . Berry’s phase is a quantum-mechanical phenomenon that may be observed at the macroscopic optical level through the use of an enormous number of photons in a single coherent state [22] . A direct macroscopic measurement of Berry’s phase may be obtained through an observation of the polarization rotation of plane-polarized light when it is transported along a closed path in momentum space [23] . Few experiments on the manifestations of Berry’s phase for photons have been reported, and those that have been can be divided into those that use optical fibre [23] , [24] , [25] and those that use discrete optical components [26] , [27] . The angle of rotation of the polarized light does not come from a local elasto-optic effect caused by torsional stress and the effect is independent of detailed material properties. The rotation angle arises only from the overall geometry of the path taken by the light. It is a global topological effect [23] . In the special case of planar (non-helical) paths, such as the paths typically taken by planar optical waveguides, no significant optical rotation is observed independent of the complexity of the path [23] . The key to manifest Berry’s phase in photonic integrated circuits is to introduce out-of-plane three-dimensional waveguides to create a two-dimensional momentum space with non-zero (Gaussian) curvature. Accessing Berry’s phase on a silicon chip We introduce the physical waveguide layout shown in Fig. 1a and its momentum space in Fig. 1b . Monochromatic light at wavelength λ carries a momentum given by , where k is the propagation vector with magnitude 2 π / λ and ħ is the Planck’s constant divided by 2 π . In physical space, the layout consists of three main portions. The first portion, shown in red in Fig. 1a , consists of an ascending out-of-plane 180° waveguide bend. The second portion, shown in green, consists of an out-of-plane waveguide that descends to the chip surface. Finally, the third portion consists of an in-plane 180° bend. In momentum space, the corresponding paths for each waveguide portion are shown in Fig. 1b . Light propagation along the three-dimensional path in physical space results in a non-zero subtended solid angle in momentum space, shown as the shaded area in Fig. 1b . Therefore, the waveguide geometry will exhibit Berry’s phase. A change in wavelength results in a change of the radius of the sphere in momentum space but not the solid angle. Therefore, the effect is intrinsically broadband. If the deflection angle of waveguide portion 1 in the physical space shown in Fig. 1a is θ , then the output light will appear with polarization rotation equal to 2 θ due to Berry’s phase because the magnitude of the solid angle extended by the grey area in momentum space, shown in Fig. 1b , is 2 θ . 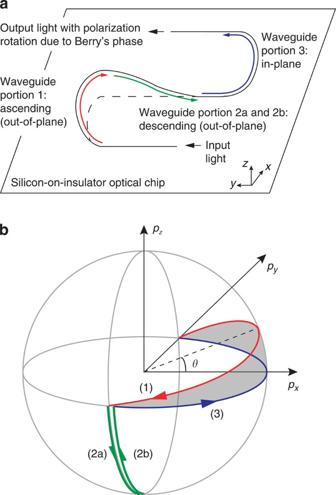Figure 1: Concept to realize Berry’s phase in silicon photonic integrated circuits. (a) Physical space: waveguide layout involving out-of-plane waveguides. (b) Momentum space: non-zero solid angle subtended by the shaded surface corresponds to the Berry’s phase which, manifests as polarization rotation. The numbers in parentheses correspond to paths in physical space ina. Figure 1: Concept to realize Berry’s phase in silicon photonic integrated circuits. ( a ) Physical space: waveguide layout involving out-of-plane waveguides. ( b ) Momentum space: non-zero solid angle subtended by the shaded surface corresponds to the Berry’s phase which, manifests as polarization rotation. The numbers in parentheses correspond to paths in physical space in a . 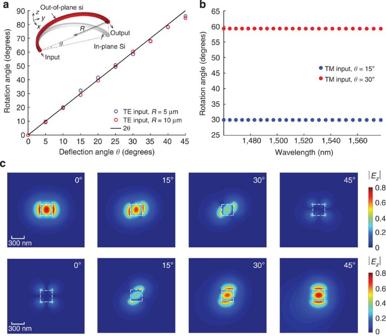Figure 2: Finite difference time domain modeling of optical polarization rotation from Berry’s phase. (a) Rotation angle versus deflection angle with bend radius as parameter for TE polarized input light at 1,550 nm wavelength. Inset: schematic of out-of-plane waveguide in computational domain. (b) Rotation angle versus wavelength with deflection angle as parameter for TM polarized input light. (c) Waveguide mode at 1,550 nm wavelength for deflection angle equal to 0°, 15°, 30° and 45° in sequence. The silicon waveguide core cross-section is 300 × 300 nm. The core is clad in silicon dioxide on all sides. Full size image Numerical modelling Figure 2 shows the results of numerical simulation of polarization rotation due to the out-of-plane 180° silicon waveguide bend using finite difference time domain computations at 1,550 nm wavelength. The geometry for the simulation domain is shown in the inset of Fig. 2a . Figure 2a shows the polarization rotation of transverse electric (TE) polarized input light versus vertical deflection angle θ for bend radii R equal to 5 and 10 μm. The simulated polarization rotation angle is in good agreement with 2 θ . The polarization rotation angle does not change with radius because the solid angle 2 θ is constant with radius. Figure 2b shows the polarization rotation angle of transverse magnetic (TM) polarized input light versus wavelength for θ equal to 15 and 30°. The polarization rotation is weakly dependent of wavelength, with less than 0.2° variation from 1,460 to 1,580 nm. For TE input polarization at 1,550 nm wavelength, Fig. 2c shows the output electrical fields of the waveguide mode horizontal component, E y , and vertical component, E z , for θ equal to 0°, 15°, 30° and 45° (see Supplementary Note 1 ). The corresponding polarization rotation angles are 2 θ . Figure 2: Finite difference time domain modeling of optical polarization rotation from Berry’s phase. ( a ) Rotation angle versus deflection angle with bend radius as parameter for TE polarized input light at 1,550 nm wavelength. Inset: schematic of out-of-plane waveguide in computational domain. ( b ) Rotation angle versus wavelength with deflection angle as parameter for TM polarized input light. ( c ) Waveguide mode at 1,550 nm wavelength for deflection angle equal to 0°, 15°, 30° and 45° in sequence. The silicon waveguide core cross-section is 300 × 300 nm. The core is clad in silicon dioxide on all sides. Full size image Design and experiment In fabricated devices, deflection angles larger than a few degrees are challenging to achieve. Therefore, for a first proof-of-concept experiment, a compact microring cavity with small deflection angle is utilized to accumulate polarization rotation over multiple round trips [25] , [28] . The narrow band spectral features of the ring resonator superimpose on the broadband polarization rotation from Berry’s phase. A schematic of the out-of-plane ring cavity is shown in Fig. 3a . The out-of-plane portion of the ring consists of a waveguide bend and an inclined straight section. The out-of-plane deflection is produced by thin film stress in the silicon dioxide bilayer. Light is coupled to the ring by a Mach–Zehnder coupling region with a Ti microheater for thermo-optic control of waveguide-coupled feedback [29] , [30] , [31] . Electrical tuning enables dynamic control of the polarization rotation. Fig. 3b shows a top–down optical micrograph of the fabricated device. The out-of-plane ring radius is 20 μm and the straight sections are 40 μm in length. The vertical out-of-plane deflection is 1 μm, measured by optical interferometric surface profilometry and shown in Fig. 3c . The ring-to-bus coupling gaps are 100 nm to enable strong coupling [29] , so that the outer 343.4 μm optical path dominates the optical resonance characteristics. To characterize the polarization rotation, the output bus waveguide is connected to an on-chip TE–TM polarization splitter with 10 dB polarization extinction ratio in the optical C band [32] . D.C. electrical power is applied to the thermo-optic heater from 0 to 76 mW in increments of 4 mW. Additional fabrication and measurement details are given in the Methods. 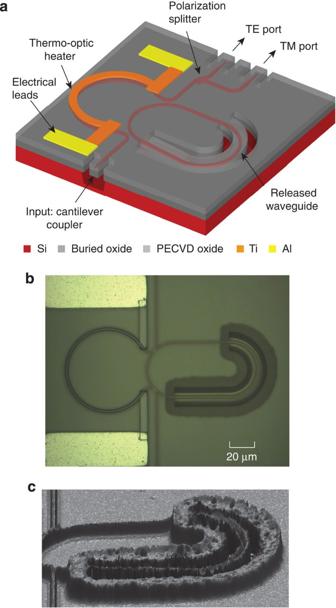Figure 3: Electrically tunable polarization rotation. (a) Schematic of device. (b) Top–down optical micrograph of fabricated device. (c) Optical interferometric surface profilometer measurements of out-of-plane waveguide. The silicon waveguide core bottom width is 310 nm and the height is 300 nm (seeSupplementary Fig. 1). The sidewall angle is 86°. Figure 3: Electrically tunable polarization rotation. ( a ) Schematic of device. ( b ) Top–down optical micrograph of fabricated device. ( c ) Optical interferometric surface profilometer measurements of out-of-plane waveguide. The silicon waveguide core bottom width is 310 nm and the height is 300 nm (see Supplementary Fig. 1 ). The sidewall angle is 86°. Full size image Measurements and characterization The optical transmission spectra for TE input light as a function of wavelength and applied electrical power P to the thermo-optic heater are shown in Fig. 4 . Due to the phase tuning of the feedback arm, the polarization state and the resonance wavelength are tuned simultaneously. Coupling between TE and TM modes produce optical transmission lineshapes that evolve from a single notch, to two separate notches, and then back to a single notch over the range of electrical powers shown (see Supplementary Note 1 , Supplementary Figs 2 and 3 ). 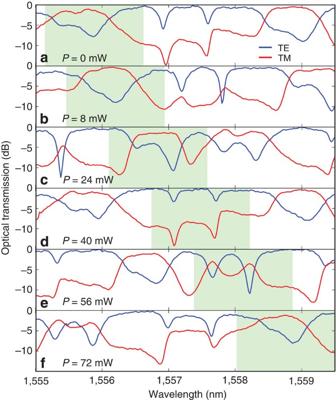Figure 4: Optical transmission measurements. The input optical polarization is TE. Green-colored windows indicate a full free spectral range of identical resonance order. Electrical powerPdynamically converts the optical polarization from TE to TM. Blue curve indicates TE polarization. Red curve indicates TM polarization. Panelsatofindicate optical transmission measurements with six different applied electrical powersP. Figure 4: Optical transmission measurements. The input optical polarization is TE. Green-colored windows indicate a full free spectral range of identical resonance order. Electrical power P dynamically converts the optical polarization from TE to TM. Blue curve indicates TE polarization. Red curve indicates TM polarization. Panels a to f indicate optical transmission measurements with six different applied electrical powers P . Full size image The polarization conversion efficiency is highest at the resonance wavelengths. In Fig. 4 , a green-coloured window is used to track a full free spectral range of identical resonance order for each value of electrical power as the resonance wavelength is tuned at a rate of 0.04 nm mW −1 . Comparing Fig. 4a,f , we observe that the free spectral range window for the same resonance order exhibits a similar spectrum, indicating that the electrical power required to achieve a 2 π optical phase shift in the feedback arm is approximately 72 mW. In Fig. 4b , the local minimum at 1,556.2 nm corresponds to a TE resonance with 9 dB transmission extinction ratio. We observe nearly complete conversion from TE input polarization to TM output polarization. Comparing Fig. 4b,d , the TM-to-TE polarization extinction ratio (PER= P TM / P TE ), dynamically changes from +9 dB at 1,556.2 nm in Fig. 4b to −10 dB at 1,557.48 nm in Fig. 4d , with less than 1 dB conversion loss. The loss is attributed primarily to propagation loss. 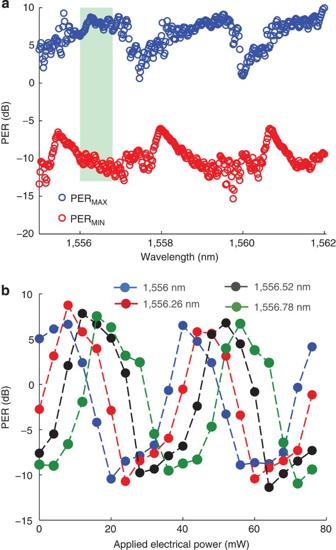Figure 5: Measurements of polarization extinction ratio. (a) Maximum and minimum polarization extinction ratio versus wavelength for a specific electrical power. (b) PER versus electrical power with wavelength as parameter. Continuous tuning between TE and TM optical polarization is observed. Wavelengths are selected from green shaded region ina. Figure 5a presents maximum PER, denoted PER MAX , and minimum PER, denoted PER MIN , versus wavelength for a specific electrical power in the range from 0 to 76 mW. The maximum to minimum PER can be as large as 21.4 dB. The PER versus electrical power at four specific wavelengths is shown in Fig. 5b . For each wavelength, the PER is observed to be continuously tunable between TM and TE polarizations. Figure 5: Measurements of polarization extinction ratio. ( a ) Maximum and minimum polarization extinction ratio versus wavelength for a specific electrical power. ( b ) PER versus electrical power with wavelength as parameter. Continuous tuning between TE and TM optical polarization is observed. Wavelengths are selected from green shaded region in a . Full size image Our demonstration of electrically controllable optical polarization rotation utilizing Berry’s phase in silicon photonics establishes new horizons for the dynamic control of optical polarization on the chip-scale. In addition to polarization rotators, dynamic control of optical polarization rotation can be utilized to realize a new class of components in integrated photonics including polarization mode modulators, multiplexers, filters and switches for advanced optical signal processing, coherent communications and sensing. Furthermore, a cascade of out-of-plane waveguides can be designed to yield broadband polarization rotation without the bandwidth constraints of a resonant ring structure. Dynamic control of optical polarization can then be achieved by tuning the deflection angle of the out-of-plane waveguides by mechanisms such as the electrostatic [33] or piezoelectric effects [34] . Fabrication Devices were fabricated on a silicon-on-insulator wafer with a 300-nm thick silicon device layer and 1 μm of buried oxide (BOX). Silicon waveguides were patterned by electron-beam lithography using an HSQ mask and etched by Cl 2 /O 2 reactive ion etching [35] . A top cladding of silicon oxide was deposited using plasma enhanced chemical vapour deposition to a thickness of 1 μm. The microheater consists of 150 nm thick titanium and 250 nm thick aluminium electrical pads, deposited by electron-beam evaporation and sequentially patterned using a lift-off process. Pad-to-pad metal resistance was measured to be 2.8 kΩ. A 300-nm thick PECVD oxide was then deposited to passivate the metal. A 200-nm Cr film was then evaporated and 300-nm PECVD oxide was deposited for electron-beam lithography writing to form a Cr mask for SF 6 RIE release of the out-of-plane portion of the ring and the cantilever couplers [36] , [37] . The Cr mask was etched by wet chemistry before device characterization. Measurement setup To experimentally characterize the on-chip polarization rotation, light from an off-chip tunable infrared continuous-wave laser is connected to a fibre polarization controller that produces linearly polarized TE light with a cross polarization extinction ratio of 16 dB. Tapered fibres are used for fibre-to-chip coupling using cantilever couplers [36] , [37] . Output light from the on-chip polarization splitter is collected to a photodetector and measured with a power meter. The optical transmission measurements are normalized by the off-resonance TE power. How to cite this article : Xu, Q. et al. Electrically tunable optical polarization rotation on a silicon chip using Berry’s phase. Nat. Commun. 5:5337 doi: 10.1038/ncomms6337 (2014).